Super-resolution surface mapping using the trajectories of molecular probes The surface characterization of 'soft' materials presents a significant scientific challenge, particularly under 'wet' in situ conditions where a wide variety of non-covalent interactions may be relevant. Here we introduce a new chemical imaging method, MAPT (mapping using accumulated probe trajectories) that generates images of surface interactions by distributing different aspects of molecular probe trajectories into distinct locations and then combining many trajectories to generate spatial maps. The maps are super-resolution in nature, because they are accumulated from highly localized single-molecule observations. Unlike other super-resolution techniques, which report only photon or point counts, our analysis generates spatial maps of physical quantities (adsorption rate, desorption probability, local surface diffusion coefficient, surface coverage/occupancy) that are directly associated with the molecular interactions between the probe molecule and the surface. We demonstrate the feasibility of this characterization using a surface patterned with various degrees of hydrophobicity. Surface modification has become a critical component of micro- and nanofabrication with applications in technologies ranging from biodetection [1] , [2] to catalysis [3] , [4] and many more [5] , [6] , [7] , [8] . Many of these applications exploit non-covalent interactions and molecular recognition. In contrast with the situation for 'hard' materials in vacuo , where numerous analytical methods exist to detect and map atomic species, there is a dearth of appropriate characterization methods for 'soft' molecular materials, where non-covalent molecular interactions are paramount, and applications often involve 'wet' conditions. Methods based on scanning probe microscopy (SPM, for example, chemical force microscopy [9] , [10] , [11] ) can provide some local information about surface interactions. However, SPM has significant limitations in this regard, not the least of which is the need to understand the surface chemistry of the probe tip itself. In addition, the time resolution of SPM is poor and there are severe challenges with respect to the robustness and reproducibility of probe chemistry. In recent years, super-resolution optical microscopy methods have been developed that compile accumulated observations of individual molecules to create images with resolution beyond the diffraction limit. STORM [12] (stochastic optical reconstruction microscopy) and PALM [13] (photoactivated localization microscopy) are perhaps the best-known examples. PAINT [14] (point accumulation for imaging in nanoscale tomography) is a similar approach that has been applied at surfaces, using randomly adsorbed molecules from solution to identify surface features with super-resolution precision [14] , [15] , [16] , [17] . This is a powerful concept; however, the methods developed to date provide images that are based purely upon 'point counts' (a relative contrast mechanism) and lack the general ability to connect observed features with specific material properties and interactions. In addition, these techniques are thus far limited to special cases of complementary DNA [15] on surfaces, local surface enhancement from hotspots [17] or where the surface selectively quenches fluorescence outside features of interest [14] , [16] . Our goal here is to develop a generally applicable super-resolution surface mapping method, where features observed in images can be directly related to specific surface functionalities. In previous work, we demonstrated the ability of single-molecule total internal reflection fluorescence microscopy (TIRFM) to quantify the adsorption [18] , [19] and diffusion [19] , [20] , [21] of surfactant probes at the solid–liquid interface in an effort to understand fundamental dynamic interfacial behaviour. In this paper, we turn this approach upside down, and use the trajectories of probe molecules (BODIPY-labelled dodecanoic acid) to provide images based on the lateral heterogeneity of probe–surface interactions. Importantly, we use the absolute physical properties of these interactions to map a surface, rather than arbitrary photon or point counts. We call this new approach mapping using accumulated probe trajectories (MAPT). To implement mapping based on the dynamic details of molecular trajectories, an enormous leap was required in terms of the number of trajectories analyzed, from ~10 2 , in a typical single-molecule tracking experiment, to 10 5 –10 6 . This was achieved by developing efficient, high-throughput computational methods, which enabled us to extract quantitative information from massive data sets. After obtaining maps of several dynamic probe properties (adsorption rate, interfacial mobility, occupancy, desorption probability), we directly relate these physical properties back to 'calibration' data from uniform surfaces to identify the specific hydrophobicity associated with each region. This demonstration system (where hydrophobic interactions are the dominant interaction) allows us to make direct connections between standard macroscale measurements of hydrophobicity (contact angle) and small-scale probe–surface interactions of the MAPT technique. We also demonstrate that spatial features can be identified at super-resolution length scales. MAPT images of hydrophobicity Recent molecular simulations have suggested that single-molecule interactions can potentially identify nanoscale differences in hydrophobicity [22] . Here, we use a photo-patterned hydrophobically modified surface [23] as a model system to prepare spatially well-defined areas of varying hydrophobicity, and a fluorescently labelled fatty acid (BODIPY-labelled dodecanoic acid) as a probe molecule. Fatty acid surfactants are good model systems for studying hydrophobic interactions in aqueous interfacial systems—in part due to the carboxyl group, which enhances water solubility through hydrogen bonding, and to the alkyl tail that remains largely unsolvated in an aqueous phase, while retaining sufficient solubility. BODIPY is one of the most hydrophobic fluorophores available, hence it is also particularly appropriate for these experiments. Consistent with these expectations, previous experiments that measured activation energies associated with the surface diffusion of BODIPY-labelled fatty acids [21] , and images based on probe–surface affinity [23] suggested that this homologous series of probe molecules interacted with trimethylsilyl (TMS)-coated fused silica (FS) primarily via hydrophobic interactions. To demonstrate the utility of MAPT, we created a patterned TMS surface using ultraviolet photodegradation. The sample surface was exposed to ultraviolet light for 180 s with a TEM grid as a contact mask. To put this into context, 180 s of photodegradation reduced the water contact angle of a homogeneous TMS surface from ~94° to ~69°. The surface was exposed to a solution of BODIPY-dodecanoic acid at concentrations of 10 −12 to 10 −15 M. These concentrations are sufficiently low that no significant self-assembly occurs on the surface. In fact, except for a tiny fraction of photobleached molecules, we can explicitly see each molecule adsorbed on the surface, and the average fractional surface coverage is typically on the order of 10 −9 . 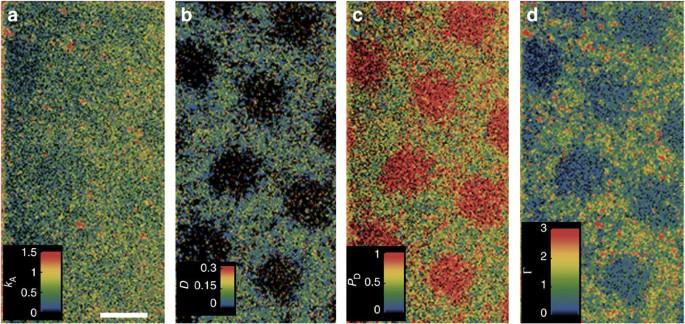Figure 1: MAPT images of the photopatterned TMS surface. MAPT images of (a) adsorption ratekA(1013μm−2s−1M−1) (b) average diffusion coefficientD(μm2s−1) (c) desorption probability per 400 msPDand (d) surface coverage/occupancy Γ (1013μm−2s−1M−1) on a photo-patterned TMS surface. Scale bar, 10 μm ina. Figure 1 shows MAPT images of the photo-patterned TMS surface that are based on the adsorption rate, average diffusion coefficient, desorption probability and occupancy (that is, mean surface coverage) of the surface. The bin (that is, pixel) size for these images was 270×270 nm. All four images were extracted simultaneously from the same ~330,000 probe trajectories. The pattern associated with the photomask is clearly visible in all four MAPT images. In particular, square regions associated with the less hydrophobic photodegraded areas are visible, surrounded by more hydrophobic undegraded regions. In Figure 1a , the adsorption rate is greater (red, yellow, green) in the hydrophobic areas, whereas the adsorption rate is lower (blue, green) in the degraded regions. In Figure 1b , one sees slower probe diffusion (green, blue) in the undegraded regions and faster diffusion (red, yellow) within the degraded regions. There is also a significant amount of black (that is, empty pixels corresponding to no displacements), which is a consequence of the lower overall adsorption rate and the high probability of desorption seen in Figure 1c . In Figure 1c , the hydrophobic areas have a lower probability of desorption (blue, green, yellow), whereas in the less hydrophobic regions mostly red pixels are observed, which correspond to a high probability of desorption. Figure 1d shows that the surface coverage in the hydrophobic areas is significantly higher (red, yellow, green) than in the hydrophilic regions (blue, black). Figure 1: MAPT images of the photopatterned TMS surface. MAPT images of ( a ) adsorption rate k A (10 13 μm −2 s −1 M −1 ) ( b ) average diffusion coefficient D (μm 2 s −1 ) ( c ) desorption probability per 400 ms P D and ( d ) surface coverage/occupancy Γ (10 13 μm −2 s −1 M −1 ) on a photo-patterned TMS surface. Scale bar, 10 μm in a . Full size image In addition to the overall trend observed in the various dynamic probe behaviours, local variation is also clearly observed on μm length scales within both the degraded and undegraded regions. The cross-correlation of various properties provides strong evidence that this spatial variation is representative of actual material properties. For example, in the undegraded TMS regions, we see many small (submicron) regions of high adsorption (bright red regions in Fig. 1a ) that also correspond to areas of high occupancy (colocalized red spots in Fig. 1d ), lower desorption probability (blue spots in Fig. 1c ) and slower interfacial diffusion (green or blue in Fig. 1b ). These features persist across independent measurements of the surface, indicating that they are not merely statistical artifacts, but real surface features. The 'hotspots' have not been seen in atomic force microscopy (AFM) images [23] of TMS or photodegraded TMS surfaces. Many of these small features on these maps also contain interesting substructure, which can be accessed by decreasing the size of the bins. The resolution limits of such substructures will be explored later in the letter. An important experimental consideration is the effect of photobleaching on the MAPT desorption probability image. We can place a lower limit on the characteristic timescale for photobleaching using the longest-lived molecular population. On TMS, this is measured to be 14.5±1.4 s, which corresponds to a desorption probability of 0.028±0.003. In the context of MAPT imaging, this represents a background level in the desorption probability channel, and it is an order of magnitude lower than any desorption probability seen in the maps. Surface roughness from the photodegradation might be expected to contribute to both the overall trends in dynamics, as well as the 'hotspots'. However, in previous work [24] , the primary source of surface roughness was determined to be from the FS substrate, not from the photodegredation of the TMS layer. Therefore, the surface chemistry would seem to be the dominant factor for the trends in overall dynamics, as well as the 'hotspots'. Chemical identification The fact that the details of the contrast in the images in Figure 1 can be directly related to actual physical phenomena provides deep insight into the local probe–surface interactions. However, the ultimate goal of MAPT is to go beyond this, and to directly identify regions of an image with a particular surface chemistry. This is possible because the numerical values comprising the MAPT images are not arbitrary, but rather represent absolute values of measurable physical properties. Therefore, one can separately perform calibration experiments on unpatterned surfaces of known surface chemistry, and compare the corresponding values of dynamic parameters to local values in MAPT images. 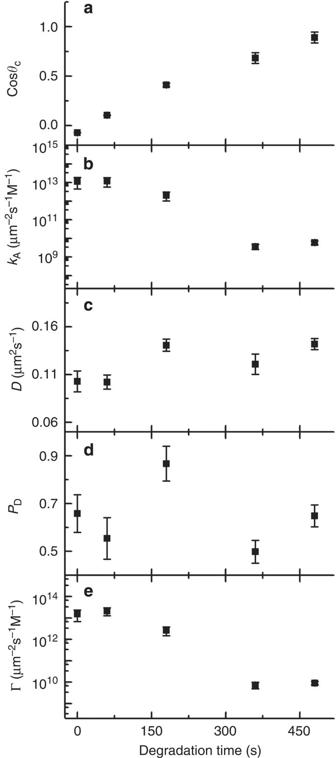Figure 2: Characterization data from homogenous TMS surfaces versus ultraviolet degradation exposure. (a) Cosine of the contact angleθc, (b) adsorption ratekA, (c) average diffusion coefficientD, (d) desorption probability per 400 msPD, (e) surface coverage Γ (that is, occupancy). Error bars represent the standard deviation from replicate measurements. Figure 2 shows an overview of the values obtained in such calibration experiments, where parameters of mean adsorption rate, surface diffusion coefficient and so on were measured on unpatterned TMS surfaces that had been photodegraded for various lengths of time. In addition, Figure 2a shows the contact angle on these surfaces, specifically the increase in cos( θ c ) with degradation time, where θ c is the static contact angle of water on the surface under ambient conditions. In previous work [24] , we have shown that the static, receding and advancing contact angle for undegraded and photodegraded TMS surfaces are equivalent within experimental uncertainty. This trend shows a transition from a hydrophobic surface for pure TMS to a hydrophilic surface at long degradation times, with the contact angle at 480 s matching the expected contact angle for water on a FS surface. Although some of the properties vary in a smooth and intuitive way with increased degradation time, others exhibit unexpected non-monotonic behaviour, which we hypothesize may be related to nanoscale heterogeneity introduced by the photodegradation process. We emphasize that the main purpose of these data in the context of this manuscript is to obtain a characteristic 'fingerprint' of a given type of surface in terms of dynamic probe properties. Figure 2: Characterization data from homogenous TMS surfaces versus ultraviolet degradation exposure. ( a ) Cosine of the contact angle θ c , ( b ) adsorption rate k A , ( c ) average diffusion coefficient D , ( d ) desorption probability per 400 ms P D , ( e ) surface coverage Γ (that is, occupancy). Error bars represent the standard deviation from replicate measurements. Full size image In Figure 2b the average adsorption rate k A is observed to decrease rapidly by nearly three orders of magnitude over the range of the degradation times measured. It is important to note that this is the rate of individual molecules adsorbing to the surface, not the macroscopic net absorption rate that is measured using ensemble-averaging methods. The average diffusion coefficient, D , increases gradually with decreasing hydrophobicity ( Fig. 2c ), but varies in an irregular way in intermediate ranges. The average desorption probability, P D , also exhibits non-monotonic behavior with a clear maximum at 180 s degradation time ( Fig. 2d ). Figure 2e shows the average surface coverage, Γ, which is conceptually related to the competition between adsorption rate and desorption probability; this quantity decreases rapidly with degradation time ( Fig. 2e ). These data collectively show how fatty acid probe interactions ( Fig. 2b–e ) change with increasing photodegradation of TMS surfaces, and form a basis for correlating the local quantities obtained from MAPT image sets with macroscopic properties such as hydrophobicity. 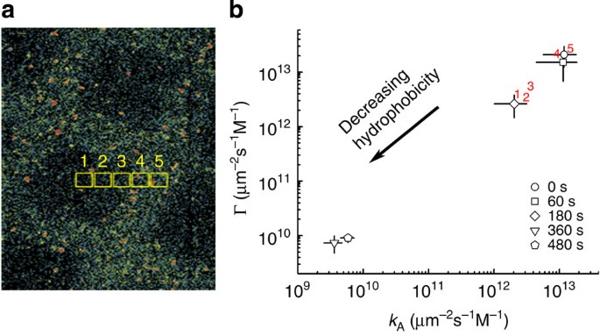Figure 3: MAPT image regions compared with data for homogenous TMS surfaces. (a) Spatial map of adsorption on a TMS surface patterned by ultraviolet light for 180 s with the regions of interest marked by yellow squares and labelled with corresponding identification numbers. (b) Surface coverage (Γ) versus adsorption rate (kA) from the homogenous surface measurements (plotted with symbols) and the regions of interest (plotted with numbers corresponding to the region of interest inFig. 3a). To make direct connections between MAPT images in Figure 1 and the calibration data in Figure 2 , we chose several regions of interest that are marked in Figure 3a as numbered yellow squares. Regions 1–3 are in photodegraded areas, whereas regions 4 and 5 are in areas that were protected by the photomask. Figure 3b compares the mean values of surface coverage/occupancy and adsorption rate from both the homogenous surface measurements (plotted with symbols) and the regions of interest (plotted with numbers corresponding to the region of interest in Fig. 3a ). Figure 3: MAPT image regions compared with data for homogenous TMS surfaces. ( a ) Spatial map of adsorption on a TMS surface patterned by ultraviolet light for 180 s with the regions of interest marked by yellow squares and labelled with corresponding identification numbers. ( b ) Surface coverage (Γ) versus adsorption rate ( k A ) from the homogenous surface measurements (plotted with symbols) and the regions of interest (plotted with numbers corresponding to the region of interest in Fig. 3a ). Full size image In Figure 3b , the values of both adsorption rate and occupancy for regions 1 and 2 are within experimental uncertainty of the values associated with the homogenous surface degraded for 180 s (diamond). Similarly, the values of both parameters for regions 4 and 5 are within experimental uncertainty of the values associated with the undegraded TMS surface (circle). Interestingly, region 3 exhibits values of the adsorption rate and surface occupancy that are intermediate between the values associated with homogeneous surfaces degraded for 60 s (square) and 180 s (diamond), suggesting that region 3 corresponds to a location with an intermediate hydrophobicity. This is expected given its location near the edge of the degraded region. Such hydrophobicity gradients have been previously observed [24] and correlated with novel nanoparticle dynamics. This analysis demonstrates that we can make calibration measurements of absolute physical quantities on homogenous surfaces and then match these quantities to the measured properties of regions on heterogeneous surfaces. In effect, single-molecule interactions can be used to probe local hydrophobicity quantitatively on an absolute scale. Super-resolution imaging Thus far, we have demonstrated that MAPT can be used to identify heterogeneity of surface chemical functionality on length scales of ~0.5–20 μm. However, because the MAPT approach involves the accumulation of single-molecule trajectories, it is inherently capable of resolving features that are smaller than the diffraction limit. Figures 4a and c demonstrate the super-resolution capabilities of MAPT using two representative surface maps of surface coverage, which are on TMS surfaces that had been degraded for 360 and 210 s, respectively. 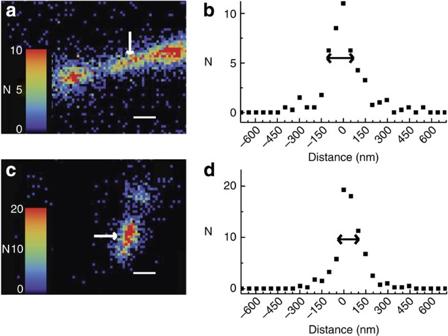Figure 4: MAPT images with line scan graphs demonstrating super-resolution. Surface coverage maps of small features on a TMS surface degraded for 360 s (a) and a TMS surface degraded for 210 s (c) with corresponding cross-sections of the surface coverage in number of molecules (N) showing the full width, half maximum (indicated by the double arrows) of (b) 175 nm and (d) 125 nm. Scale bars, 500 nm ina,c. Figures 4b and d show corresponding line scans associated with the arrows in Figure 4a and c , respectively. In these examples, we use the full-width at half-maximum (FWHM) of the indicated features to estimate the width of the surface feature. The apparent width of the feature in Figure 4b is 175 nm and in Figure 4d is 125 nm, which are significantly below the diffraction limit (~300 nm). Figure 4: MAPT images with line scan graphs demonstrating super-resolution. Surface coverage maps of small features on a TMS surface degraded for 360 s ( a ) and a TMS surface degraded for 210 s ( c ) with corresponding cross-sections of the surface coverage in number of molecules ( N ) showing the full width, half maximum (indicated by the double arrows) of ( b ) 175 nm and ( d ) 125 nm. Scale bars, 500 nm in a , c . Full size image The ultimate resolution limits for super-resolution techniques depend on many factors [25] , including the interfacial mobility of the molecules, the frame acquisition time, the signal to background ratio of the fluorescent emission from single molecules, the number of molecules, compensation for mechanical drift and the details of the calculation of the centre of intensity. Using the PAINT technique, resolution limits of 18 nm have been reported [16] , and MAPT is fundamentally capable of producing similar results under the same experimental conditions. In our experiment, the long acquisition time (400 ms), lack of compensation for mechanical drift and mobility of the molecules are the primary sources of the relatively large resolution limit (125 nm), in comparison with similar experiments (18 nm). Although faster acquisition time and mechanical drift can be corrected for by modification of the experimental setup, the mobility of the molecules likely represents a fundamental limitation of spatial resolution (from point spread function broadening) of the MAPT technique. The probe mobility also provides advantages, however, because mobile probe molecules 'explore' large areas of the surface, which enhances the molecular targeting of any rare, small-scale surface features. Here we demonstrate that even using mobile single surfactant molecules on a general hydrophobic surface (without quenching to enhance contrast), it is possible to map features with super-resolution. The MAPT technique provides spatial maps, based on unique in-situ molecular-probe dynamics that are distinct from and complementary to images obtained using preexisting methods, for example, scanning probe microscopy. In principle, the MAPT technique could reach the same probe densities as AFM/scanning tunneling microscopy measurements, given enough molecules on the surface, which is mainly a matter of increasing the total time of trajectory accumulation. In practice, however, to reach such high densities would require a number of single-molecule localizations that is not currently computationally feasible. Thus, the practical resolution limit for the MAPT technique is likely similar to other techniques that rely on random adsorbing molecules, which is an order of magnitude greater than typical AFM experiments. The contrasting nature of length scales and measurement versatility show that the MAPT technique is not a replacement for AFM/scanning tunneling microscopy, but is rather a complementary technique. Interestingly, the actual contrast precision and resolution of MAPT images are not purely a function of the total number of accumulated trajectories. For example, even with a large overall density of molecular trajectories in Figure 1 , the diffusion coefficient map ( Fig. 1b ) exhibits low density within the photodegraded areas. This is due to the very short residence times in those surface regions, which results in short local trajectories. This demonstrates an interesting feature of this method: because we are exploiting intrinsic dynamic interfacial phenomena of the adsorbate molecules to prepare these maps, for a given probe–surface combination, certain contrast mechanisms will typically provide greater contrast and/or resolution than others. By exploiting a wide range of different combinations of probe chemistry, solvent and surface, our expectation is that the MAPT technique will be able to visualize and identify many varied surface chemistries. It is interesting to speculate on possible applications of MAPT to other examples of surface chemistry heterogeneity. For example, single-molecule imaging was recently used to show a lack of spatial correlations for chemical reactions on a surface [26] . Using MAPT for a similar system, one could quantify absolute chemical reaction rates on surfaces. Furthermore, using single-molecule fluorescence resonance energy transfer, conformation changes in large molecules (such as polymers or proteins) could be linked to spatial heterogeneities in surface chemistry. Lipid bilayers would also be a useful system for surface mapping, where heterogeneities in mobility could be used to both probe the structure of the bilayer and correlate novel dynamics of membrane proteins with these features. In conclusion, we have developed a new chemical imaging method based on accumulating single-molecule trajectories to generate molecular-interaction maps of surfaces. We demonstrated that this mapping technique could be used to quantify spatially heterogeneous average physical quantities associated with hydrophobicity and then identify the specific contact angles associated with those regions using calibration data from uniform surfaces. We also showed that these maps are capable of identifying spatial heterogeneities on super-resolution length scales. Sample preparation Surfaces were prepared by photodegradation of hydrophobically modified FS surfaces [23] . A 50-mm diameter FS wafer (MTI Corp.) was cleaned in hot piranha solution for ~1 h followed by ultraviolet–ozone treatment for another ~60 min. The clean hydrophilic substrate was placed in a sealed glass container containing hexamethyldisilazane (HDMS, 99.8% purity, Acros Organics) and positioned ~5 cm above the liquid to expose its surface to HDMS vapour for ~48 h. In contrast with solution deposition of SAMs, this vapor-deposition process ensured that the TMS layer contained no fluorescent impurities as confirmed by control TIRFM experiments carried out with pure deionized water (Millipore, Milli-Q ultraviolet, 18.3 MΩ cm). These TMS-modified surfaces were then exposed for the desired degradation time to ultraviolet illumination from a Hg pen lamp (UVP, 254 nm) held at ~5 mm from the surface. The intensity was ~0.3 mW cm −2 at this distance. Patterning was accomplished by photodegradation using 1,500 fine grid mesh (Structure Probe Inc.) as a contact photomask. The patterned surfaces were then exposed to solutions containing fluorescently labelled dodecanoic acid (Invitrogen Bodipy FL-C 12 ) at concentrations of 10 −12 to 10 −15 M (significantly below the concentration required for self-assembly) and a time series of TIRFM images was obtained. Images for the time series were sampled continuously for 7 min, with each frame having an exposure time of 300–500 ms. Surface mapping data analysis The basis of our surface mapping method is to divide the microscope viewing area into a spatial grid divided into bins of a user-determined size (each bin serves as a pixel in the final image). The positions of all events of interest are determined for each probe molecule trajectory. These data are then sorted into the appropriate spatial bins and finally the accumulated value of each physical quantity is calculated for every bin. For example, the first position of every trajectory is defined as the adsorption location of that probe. The average local adsorption rate is therefore related to the number of molecules that adsorb within a particular bin. For consistency between experiments, the adsorption count is divided by the bin area, the total time for the experiment and by the concentration of probe molecules in solution. The scaling of the adsorption rate by the number of available probes in solution is an appropriate normalization factor for direct comparison of multiple experiments. Although the near-surface concentration would be the ideal absolute quantity to use for normalization, we cannot directly know this concentration. However, in our probe–surface system the hydrophobic interaction is dominant, and from first principles one does not expect a significant difference between the near-surface concentration and the bulk solution concentration. A similar approach is used to prepare surface maps of the mean interfacial diffusion coefficient, the desorption probability and the mean surface occupancy. Details of the algorithms for converting each component of molecular trajectories into surface maps of physical quantities will be described in detail below. 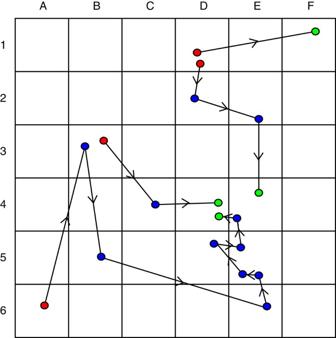Figure 5: Schematic diagram of single-molecule trajectories within a grid. First position (red), intermediate position (blue) and last position (green). Figure 5 is a schematic diagram showing several overlaid trajectories; this diagram will be used to illustrate the calculations described in the following sections. Figure 5: Schematic diagram of single-molecule trajectories within a grid. First position (red), intermediate position (blue) and last position (green). Full size image Adsorption rate Adsorption rate refers to the average number of molecules attaching to the surface per area, per time; it is also normalized by bulk concentration. This is different from the net macroscale adsorption rate, which measures the difference between the adsorption and desorption rate. The adsorption position is defined as the first position of a trajectory. The number of adsorption events for each bin is then counted. For example, in Figure 5 , bin D1 has two adsorptions, bin B3 and A6 have one adsorption each and all other bins have no adsorptions. These raw numbers are then turned into an adsorption rate by the following formula. Where N A is the number of adsorbed molecules, T is the total time, A Bin is the area per bin and C probe is the bulk solution concentration of probe. Desorption rate Desorption rate refers to the average number of molecules detaching from the surface per area, per time and bulk concentration. The desorption position is the last position of a trajectory. The number of last positions for each grid area is then counted. In Figure 5 , bin D4 has two desorption events, and bins E4 and F1 have one desorption event each. These raw numbers are then turned into desorption rate by the following formula. Where N D is the number of desorbed molecules, T is the total time and A Bin is the area per bin. Surface coverage Surface coverage (or occupancy) refers to the average number of molecules on the surface per area, per time and bulk concentration. Every recorded position of the trajectory is used to map surface coverage. The number of positions for each grid area is then counted. In Figure 5 , bin E5 has a raw occupancy of 3, bins B3, D1, D4 and E4 have raw occupancies of 2 and so on. These raw numbers are then turned into surface coverage by the following formula. Where N MP is the number of molecule positions, T is the total time, A Bin is the area per bin and C probe is the bulk solution concentration of probe. Desorption probability The desorption probability is the probability that a molecule in a given area will desorb in the next time step of the movie. For example, in Figure 5 grid E4, there is one desorption event and one molecule position from another trajectory. The desorption probability would be 0.5 because there is one desorption event divided by two molecule positions (one of which is the desorption position). The formula for this calculation is as follows. Where N MP is the number of molecule positions and N D is the number of desorbed molecules. Mean diffusion coefficient The mean diffusion is the local mean diffusion within a bin. To create a scalar map of this value, we must designate a location for the displacement vector, which is actually defined by its start and end locations. We have chosen to define the average between the start and end positions (the midpoint) as the position of the displacement. For example, a displacement occurs in Figure 5 between bins D1 and F1. Although the displacement starts in D1 and ends at F1, the displacement event will be mapped to bin E1, as this is where the midpoint of the displacement takes place. To determine an effective local diffusion coefficient, we then calculate the square of all displacements for a grid area and divide this average by four times the time per frame as described in the following formula. Where 〈Δ x 2 〉 is the mean squared displacement and t is the time per frame. The uncertainty associated with the average value of an individual bin for diffusion requires an extra term, due to the uncertainty in localizing the vector into a bin of finite size. The uncertainty for a MAPT diffusion pixel is Where σ x 2 is the uncertainty of the squared displacements, N is the number of displacements, D is the average diffusion coefficient, t is the time per frame and w is the width of the bin. The first term in the radical is for the standard error portion of the uncertainty. The second term is a ratio of average displacement to bin width, which accounts for the uncertainty in localizing the vector into a bin of finite size. Mean direction The mean direction is the local mean direction of the displacement vectors. This quantity uses the same position (midpoint of the displacement) as the mean diffusion. However, here we take the average displacement vector in a grid area and then calculate the direction of this vector. How to cite this article: Walder, R. et al . Super-resolution surface mapping using the trajectories of molecular probes. Nat. Commun. 2:515 doi: 10.1038/ncomms1530 (2011).